Travelling-wave resonant four-wave mixing breaks the limits of cavity-enhanced all-optical wavelength conversion Wave mixing inside optical resonators, while experiencing a large enhancement of the nonlinear interaction efficiency, suffers from strong bandwidth constraints, preventing its practical exploitation for processing broad-band signals. Here we show that such limits are overcome by the new concept of travelling-wave resonant four-wave mixing (FWM). This approach combines the efficiency enhancement provided by resonant propagation with a wide-band conversion process. Compared with conventional FWM in bare waveguides, it exhibits higher robustness against chromatic dispersion and propagation loss, while preserving transparency to modulation formats. Travelling-wave resonant FWM has been demonstrated in silicon-coupled ring resonators and was exploited to realize a 630-μm-long wavelength converter operating over a wavelength range wider than 60 nm and with 28-dB gain with respect to a bare waveguide of the same physical length. Full compatibility of the travelling-wave resonant FWM with optical signal processing applications has been demonstrated through signal retiming and reshaping at 10 Gb s −1 In transparent materials, the optical field interacts weakly with electrons and phonons, and thus experiences feeble nonlinear effects. Strong field confinement in nanowaveguides and materials used close to their energy bandgap are typical expedients to exploit optical nonlinearities more efficiently [1] , [2] , [3] , [4] , [5] , [6] . Further, optical resonators have been widely employed to strengthen the nonlinear interaction of optical waves and to increase the efficiency of optical parametric processes [7] , [8] , [9] , [10] , [11] , [12] , [13] , [14] , [15] . The benefit carried by light trapping in a resonator is twofold: the interaction length is enhanced with respect to the physical length by the finesse of the resonator, and the intra-cavity power is enhanced by the same factor, as a consequence of power flux conservation [10] . However, there is a price to be paid with optical resonators, and that is named bandwidth. In fact, whereas the efficiency of cavity-enhanced four-wave mixing (FWM) scales up with the cavity length, the bandwidth B scales down with it. 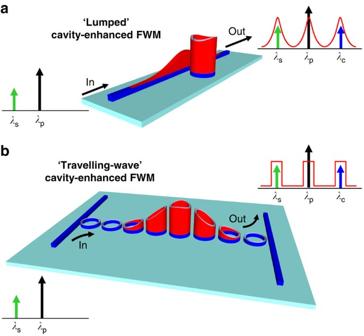Figure 1: Signal field distribution in cavity-enhanced FWM. (a) Lumped resonant FWM in a single-ring resonator. The pulse fits only partially into the single ring; (b) travelling-wave resonant FWM in a CROW. In both structures propagation and wavelength conversion are allowed only if the interacting waves lie within the passbands of the resonators, schematically illustrated by the red lines. Owing to this bandwidth-length constraint, to avoid signal distortions, the pulse length must exceed the resonator length, as shown in the schematic of Figure 1a . This implies that the resonator behaves as a concentrated device, that is, it realizes a 'lumped' nonlinear element, wherein the concept of lumped element is related to the pulse envelope rather than to its wavelength. Figure 1: Signal field distribution in cavity-enhanced FWM. ( a ) Lumped resonant FWM in a single-ring resonator. The pulse fits only partially into the single ring; ( b ) travelling-wave resonant FWM in a CROW. In both structures propagation and wavelength conversion are allowed only if the interacting waves lie within the passbands of the resonators, schematically illustrated by the red lines. Full size image The bandwidth-size constraint of cavity-enhanced FWM is not surprising. Browsing into electromagnetics textbooks, one immediately notices that this is the classical constraint people run into when dealing with lumped devices. This fundamental limitation, for example, is part of the research history of electro-optic modulators and had to be addressed in the early attempts to approach modulation speeds in the GigaHertz range. At this frequency scale, lumped electrodes were replaced by travelling-wave electrodes and this new concept enables more than one order of magnitude gain in the modulation bandwidth [16] , [17] . This analogy sounds as good news, because if a problem is not completely new, there is always some hope to find a near-at-hand solution. The question is whether it is possible to find a travelling-wave extension to the traditional concept of cavity-enhanced FWM. Travelling-wave resonant FWM would require a waveguiding structure allowing the propagation of a resonant optical field over a distance that is longer than the pulse length. The physics underlying the concept of slow light propagation in coupled-resonator optical waveguides (CROWs) fits exactly this requirement. In a CROW, the bandwidth–length constraint of the single resonator is broken, because the number of resonators can be arbitrarily increased with no bandwidth reduction [18] . As depicted in Figure 1b , the CROW length can be much longer than the pulse length, as demonstrated by recent results that reported undistorted linear pulse propagation in CROWs with a length of more than ten pulse lengths [19] . Therefore, an optical pulse travels through a CROW as in conventional waveguides, but with both enhanced power and dwelling time. The enhancement of parametric processes in CROWs was predicted nearly 10 years ago [20] , [21] , but at that time most photonic technologies were not sufficiently mature for the realization of such an advanced structure. Our recent results, demonstrating 100 Gbit s −1 linear pulse propagation [19] and nonlinear wave mixing in CROWs [22] , set a fundamental milestone in the development of this technology. In this work, we exploit nonlinear propagation in CROWs to demonstrate the new concept of travelling-wave resonant FWM. We show not only that travelling-wave resonant FWM overcomes the limits of lumped cavity-enhanced FWM, but also that the conversion process is more robust than conventional FWM against the chromatic dispersion and the propagation loss of the waveguide, while preserving entirely the intrinsic transparency to modulation formats. Nonlinear CROWs The integrated devices used in this work were fabricated in silicon-on-insulator (SOI) technology according to the procedure described in the Methods section. We used silicon photonics because it is a suitable platform to showcase the nonlinear capabilities of CROWs, but results are not restricted to a specific technology or material; other technologies employed for nonlinear processing, such as Hydex [14] , silicon nitride [15] , chalcogenide glasses [5] , [23] or silicon-organic hybrid waveguides [4] , [24] , could be used as well. 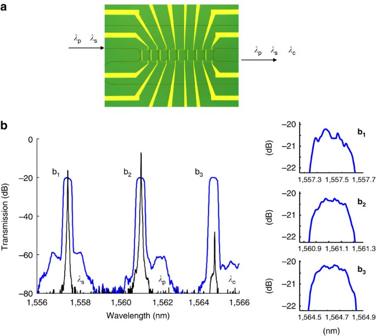Figure 2: Frequency-domain characterization of nonlinear CROWs. (a) Top-view photograph of an eight-ring CROW fabricated on an SOI platform; false colours are used to highlight the optical and the electrical structures. (b) The blue curve shows the frequency-domain response at the output port of the silicon CROW shown in (a), while the black curve shows the spectrum at the output of the CROW when pump (λp=1,561.1 nm) and signal (λs=1,557.5 nm) waves propagate inside two adjacent CROW passbands and a converted wave (λc=1,564.7 nm) is generated by travelling-wave resonant FWM inside the CROW. A detail of the CROW transmission around the signal, pump and converted wave is shown in b1, b2and b3, respectively. Figure 2a shows in a top-view photograph one of the fabricated CROWs consisting of eight identical racetrack ring resonators with radius ρ =20 μm and a straight coupling section of 16 μm. The first and the last ring are coupled to the input and output bus waveguides, respectively. The silicon nanowaveguide of the bus lines and of the rings is 220 nm high, 480 nm wide and is buried into a silicon oxide upper cladding. The waveguide propagation loss α is about 2 dB cm −1 at a wavelength of 1,550 nm. Figure 2: Frequency-domain characterization of nonlinear CROWs. ( a ) Top-view photograph of an eight-ring CROW fabricated on an SOI platform; false colours are used to highlight the optical and the electrical structures. ( b ) The blue curve shows the frequency-domain response at the output port of the silicon CROW shown in ( a ), while the black curve shows the spectrum at the output of the CROW when pump ( λ p =1,561.1 nm) and signal ( λ s =1,557.5 nm) waves propagate inside two adjacent CROW passbands and a converted wave ( λ c =1,564.7 nm) is generated by travelling-wave resonant FWM inside the CROW. A detail of the CROW transmission around the signal, pump and converted wave is shown in b 1 , b 2 and b 3 , respectively. Full size image The spectral response at the output port of the CROW is shown in Figure 2b for a transverse electric (TE) polarized input light. Propagation in the CROW is allowed only within a comb of passbands, which exhibit a bandwidth B =50 GHz (at 3 dB attenuation), a flat-top ripple-free (<0.5 dB) characteristic (see Fig. 2b 1–3 ) and a free-spectral range (FSR) of 450 GHz. The on-chip in-band insertion loss of the CROW is less than 2 dB, while the off-band light is attenuated by more than 50 dB. The accuracy of the fabrication process guarantees the proper alignment of the rings' resonances within a range of about 65 GHz (standard deviation) [25] . Post-fabrication tuning by means of independently addressable heaters placed on top of the rings was used to compensate for the resonance spread and recover the optimum spectral response of the CROWs (see the Methods section for details) [19] , [26] . Wavelength conversion in CROWs FWM in CROWs can occur effectively only if the three interacting waves propagate in the passbands of the structure [27] . The black curve in Figure 2b shows the optical spectrum at the output of the device of Figure 2a when a continuous pump and a signal wave propagate at wavelengths λ p =1,561.1 nm and λ s =1,557.5 nm, respectively. A converted wave is generated by FWM inside a third CROW passband centred at λ c =1,564.7 nm. Owing to the frequency selectivity of the CROW, the input light in the stopbands, coming for instance from crosstalk contributions and noise from optical amplifiers (visible in Fig. 2b at a power level 22 dB below the converted wave), is filtered out by the CROW, so that no spurious contributions from and to these frequencies are generated. As in conventional FWM processes, the conversion efficiency, defined as the ratio between the output converted power P c and the input signal power P s , results from the interplay of several ingredients, including material nonlinearity, pump power ( P p ) and waveguide design. When FWM takes place inside a CROW, one additional contribution is leveraged by travelling-wave resonant propagation: this contribution, hereinafter referred to as conversion enhancement with respect to a bare waveguide, is the relevant factor to be considered to evaluate the performance of travelling-wave resonant FWM. Several structures with the same FSR of 450 GHz and different bandwidth B were fabricated to investigate the enhancement factor provided by a CROW. In all the experiments reported in the paper, the pump power coupled into the silicon waveguide was 12 dBm. The FWM enhancement factor was evaluated by comparing the conversion efficiency at the output of the different structures (due to both the bus waveguide and the CROW) with the conversion efficiency of the 5-mm-long bus waveguide only, the latter amounting to P c / P s =−36 dB. 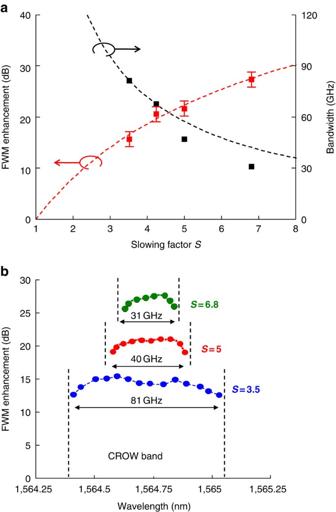Figure 3: Conversion efficiency enhancement of travelling-wave resonant FWM. (a) The red squares show the conversion efficiency enhancement of eight-ring silicon CROWs with respect to a bare waveguide with the same physical length as a function of the slowing factorS. The black squares indicate the bandwidth of the measured CROWs. The agreement with theoretical results (dashed curves) provides a direct evidence of theS4conversion gain enhancement expected in slow-light regime. (b) In-band conversion efficiency enhancement of eight-ring silicon CROWs withB=31, 40 and 81 GHz with respect to a bare waveguide with the same physical length. The almost constant conversion efficiency over the entire passband of the CROW prevents from intensity distortions of the converted wave with respect to the spectrum of the signal wave. Red squares in Figure 3a show the FWM enhancement of an eight-ring CROW with respect to a straight waveguide of the same physical length (630 μm). The corresponding CROW bandwidths are indicated by black squares. In agreement with theoretical predictions (dashed curves) [27] , experimental results show a conversion enhancement according to S 4 , where the slowdown factor S is the ratio between the group velocity of the light in a bare waveguide and the group velocity in the CROW [18] . The converted power P c is given by [27] where γ is the nonlinear propagation constant, L e is the effective nonlinear length of the CROW and η β (0< η β <1) is an efficiency parameter that includes loss and phase matching terms (see Supplementary Note 1 for details). The physical length of the CROW is L = πNρ , N being the number of rings. For a CROW with a bandwidth of about 80 GHz ( S =3.5), the enhancement factor is more than 15 dB with respect to a bare waveguide of the same length. The highest considered slowdown factor ( S =7) leads to a 28-dB enhancement, while keeping a conversion bandwidth of more than 30 GHz. In practice, the enhancement factor is limited by the maximum achievable S : at S >10 CROWs become much more sensitive to fabrication imperfections, such as non-optimum coupling coefficients between rings, resonant frequency spread [28] and roughness-induced backscattering [29] , the impact of which increases according to an S 2 dependence. Figure 3: Conversion efficiency enhancement of travelling-wave resonant FWM. ( a ) The red squares show the conversion efficiency enhancement of eight-ring silicon CROWs with respect to a bare waveguide with the same physical length as a function of the slowing factor S . The black squares indicate the bandwidth of the measured CROWs. The agreement with theoretical results (dashed curves) provides a direct evidence of the S 4 conversion gain enhancement expected in slow-light regime. ( b ) In-band conversion efficiency enhancement of eight-ring silicon CROWs with B =31, 40 and 81 GHz with respect to a bare waveguide with the same physical length. The almost constant conversion efficiency over the entire passband of the CROW prevents from intensity distortions of the converted wave with respect to the spectrum of the signal wave. Full size image With respect to FWM in single resonators, travelling-wave resonant FWM in CROWs has two remarkable advantages. The first advantage concerns the shape of the conversion band. Figure 3b shows the in-band FWM enhancement factor measured by detuning λ s across the CROW passband, while keeping the pump at a fixed wavelength λ p . Owing to the flat in-band spectral response of the CROW, the conversion band is almost flat over the entire passband, preventing from any intensity distortion. On the contrary, in single resonators both the signal and the converted waves are shaped according to a Lorentzian spectral response, resulting in a significant reduction of the conversion band. The second and more significant advantage is directly related to the travelling-wave nature of resonant FWM in CROWs. As the CROW bandwidth is independent of the number N of resonators, the length of the CROW can be increased arbitrarily, with a quadratic advantage on the nonlinear interaction. 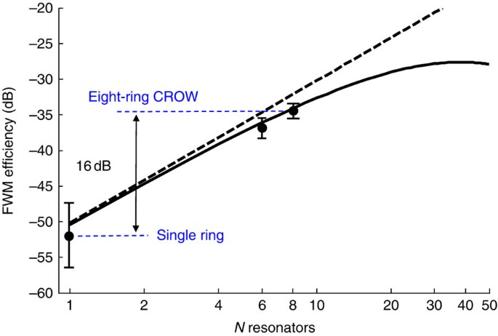Figure 4: Conversion efficiency versus the number of resonators. Marks indicate the measured conversion efficiency in a single resonator (N=1) and in CROWs with 6 and 8 coupled resonators whenPp=12 dBm. All the structures have FSR=450 GHz andB=80 GHz. The higher error bar in the measurement of the single ring is due to the extremely low conversion efficiency (<−50 dB), which is much lower than that of the 5-mm-long bus waveguide (about −36 dB). The dashed curve shows the theoretical conversion efficiency in absence of propagation loss in the CROW, whereas the solid curve takes into account 0.15 dB round trip loss in each ring of the CROW. The conversion efficiency of travelling-wave resonant FWM versus the number N of resonators is reported in Figure 4 for a silicon CROW with B =80 and FSR=450 GHz, when P p =12 dBm. Marks show the measured conversion efficiency for a single ring ( N =1) and for CROWs with 6 and 8 rings, respectively. In the eight-ring CROW, the conversion efficiency is 40 times (16 dB) higher than that provided by a single resonator of the same bandwidth and FSR. The solid and dashed curves show the theoretical conversion efficiency predicted by equation (1) in the case of null attenuation ( α =0) and 0.15 dB round trip losses within each resonator, respectively. The linear lossless curve represents the upper bound to conversion efficiency; attenuation makes the interaction efficiency reach a maximum at a finite number of cavities ( N =38) and decrease in longer structures [27] . Figure 4: Conversion efficiency versus the number of resonators. Marks indicate the measured conversion efficiency in a single resonator ( N =1) and in CROWs with 6 and 8 coupled resonators when P p =12 dBm. All the structures have FSR=450 GHz and B =80 GHz. The higher error bar in the measurement of the single ring is due to the extremely low conversion efficiency (<−50 dB), which is much lower than that of the 5-mm-long bus waveguide (about −36 dB). The dashed curve shows the theoretical conversion efficiency in absence of propagation loss in the CROW, whereas the solid curve takes into account 0.15 dB round trip loss in each ring of the CROW. Full size image Overcoming loss and dispersion limitations Travelling-wave resonant propagation enables also to push conversion efficiency beyond the well-known limits of conventional FWM. Although counterintuitive, FWM in CROWs is more robust than FWM in bare waveguides against the effects of chromatic dispersion and propagation losses, which are regarded in common belief as a serious Achilles' heel of slow-light propagation. The reason is that, according to equation (1), a CROW can be made ( S 2 +1)/2 times shorter than a bare waveguide, while keeping the same conversion efficiency. The following experiment was carried out to prove the robustness against the chromatic dispersion of the waveguide. 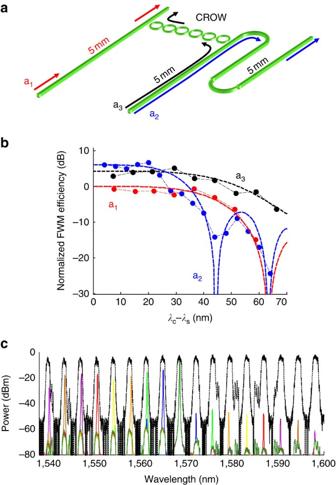Figure 5: Robustness against chromatic dispersion. (a) Schematic of the integrated circuit employed to demonstrate the benefit of travelling-wave FWM against chromatic dispersion. In cases (a1) and (a2), the pump and signal wavelengths are set off-band to avoid propagation into the CROW. (b) The maximum conversion efficiency (λc−λs≈0) of a 5-mm-long silicon waveguide (red curve, a1) is increased by lengthening the waveguide to 10-mm (blue curve, a2) or by cascading a six-ring CROW withS=3.5 (black curve, a3). In the latter case the bandwidth of the process results 1.65 times wider because of the reduced physical length of the CROW. (c) Optical spectrum at the output of the device when the pump, signal and idler waves propagate (a3) in the 5-mm-waveguide before being coupled into the CROW. Figure 5a shows the schematic of the employed circuit, consisting of a six-ring silicon CROW (FSR=450 GHz, B =81 GHz, S =3.5), which provides a 15-dB conversion enhancement with respect to a waveguide with the same physical length of 480 μm (see Fig. 3 ). The CROW is coupled with a 5-mm-long bus waveguide on one side and with a 10-mm-long bus waveguide on the other side. The input port and the wavelengths ( λ p , λ s , λ c ) were chosen in such a way that the three waves propagate (a 1 ) in the 5-mm waveguide only, (a 2 ) in the 10-mm waveguide only and (a 3 ) in the CROW after propagation in the 5-mm waveguide. Figure 5b shows that, when the length of the waveguide is doubled from 5 mm (a 1 ) to 10 mm (a 2 ), the conversion efficiency for small-wavelength detuning increases by about 6 dB, but the FWM conversion range narrows by √2 (from 41 to 29 nm), as predicted by FWM theory [30] . In (a 3 ) the three waves lie within the passing bands of the CROW; in this case the contribution to conversion efficiency given by the 0.48-mm-long CROW is 5 dB, which is comparable to that of the input 5-mm-long waveguide, but with the further advantage of increasing the FWM conversion range from 29 to 48 nm. Note that structures (a 2 ) and (a 3 ) exhibit comparable insertion loss of 2 and 3 dB, respectively. The reduction in chromatic dispersion is further confirmed by the experiment in Figure 5c , where wavelength conversion at the output of the device is observed over 16 FSRs. Even though the phase mismatch term Δ β is enhanced by a factor S inside the CROW [27] , the product Δ βL is reduced by a factor ( S 2 +1)/2 S with respect to a waveguide with the same conversion efficiency, and the conversion range widens accordingly. Note that at λ c − λ s =64 nm (8 THz) the conversion process still takes place in the CROW while it completely vanishes in the 5-mm-long waveguide. Figure 5: Robustness against chromatic dispersion. ( a ) Schematic of the integrated circuit employed to demonstrate the benefit of travelling-wave FWM against chromatic dispersion. In cases (a 1 ) and (a 2 ), the pump and signal wavelengths are set off-band to avoid propagation into the CROW. ( b ) The maximum conversion efficiency ( λ c − λ s ≈0) of a 5-mm-long silicon waveguide (red curve, a 1 ) is increased by lengthening the waveguide to 10-mm (blue curve, a 2 ) or by cascading a six-ring CROW with S =3.5 (black curve, a 3 ). In the latter case the bandwidth of the process results 1.65 times wider because of the reduced physical length of the CROW. ( c ) Optical spectrum at the output of the device when the pump, signal and idler waves propagate (a 3 ) in the 5-mm-waveguide before being coupled into the CROW. Full size image Robustness against propagation loss comes from the positive balance between conversion enhancement and effective length reduction. As P c increases quadratically with the interaction length, the maximum power that can be converted by a bare waveguide scales according to 1/ α 2 , where 1/ α (2.1 cm for α =2 dB cm −1 ) is the effective length of an infinitely long waveguide. In a CROW, the maximum effective length is reduced to 1/ S α CROW [27] , but the S 4 conversion enhancement brings the loss-limited converted power to scale with a factor and thus the overall efficiency balance is far larger than 1. Although propagation loss α CROW in the CROW can be higher than α in the bare waveguide, because of radiation loss in the bends and excess loss of the directional couplers, the CROW still provides a substantial advantage provided that α CROW < αS /2. In the specific case of silicon devices, additional power-dependent loss due to parasitic nonlinear effects, such as two-photon absorption (TPA) and free-carrier absorption (FCA), may also impair the FWM conversion efficiency [1] , [13] , [31] . Such effects can be significantly reduced by introducing a reverse biased p–i–n diode structure embedded in the silicon waveguide [32] , [33] . In our work, to avoid issues strictly related to a specific technology, our experiments were conducted in a regime where TPA and FCA have negligible effects on the conversion efficiency (see Supplementary Note 2 for details). In this way, the presented results can be straightforwardly applied to a variety of TPA-free emerging technologies that are now being explored for advanced nonlinear processing applications [14] , [15] , [23] , [24] , [32] , [33] , [34] , [35] . Phase-preserving wavelength conversion in CROW To be compliant with modern optical communication systems, which are evolving towards amplitude and phase-modulated multi-level formats, travelling-wave resonant FWM is required to entirely preserve phase information, likewise conventional FWM. To demonstrate phase-preserving wavelength conversion, a 10 Gbit s −1 differential phase shift keying (DPSK) signal is coupled to the 50-GHz-bandwidth CROW of Figure 2 after being combined with a pump wave, the state of polarization of both waves being aligned with the TE waveguide mode. Details on the experimental setup are given in the Methods section. 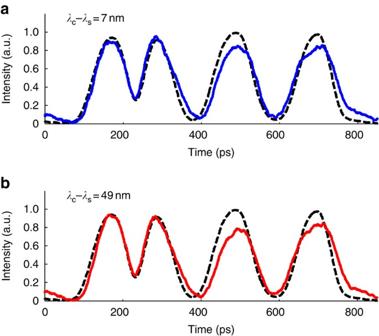Figure 6: Phase-preserving wavelength conversion in a silicon CROW. The detected bit sequence 01101010 of a 10 Gbit s−1DPSK signal at the input of a silicon CROW is shown by dashed curves, whereas the same sequence after wavelength conversion into the CROW over a wavelength rangeλc−λsof (a) 7 nm and (b) 49 nm is shown by the blue and red solid curves, respectively. The plots show the 10 Gbit s−1intensity-modulated signal detected at the output of the Mach–Zehnder delay interferometer (seeMethods). The similarity between the input (signal) and output (converted) waveforms demonstrates that no significant phase information distortion occurs. Figure 6 shows the comparison between the signal bit sequence 01101010 taken from the repetition of an 8-bit-long pattern (dashed curves) at the CROW input and the detected wavelength-converted sequence over a range λ c − λ s of (a) 7 nm and (b) 49 nm. The bit-to-bit comparison between the input (signal) and output (converted) waveforms clearly demonstrates that the phase information encoded in the original DPSK signal is well preserved with no significant quality degradation. The combination of phase preservation and in-band constant conversion efficiency (see Fig. 3b ) demonstrates that travelling-wave resonant FWM does not lose the modulation format transparency typical of conventional FWM. Figure 6: Phase-preserving wavelength conversion in a silicon CROW. The detected bit sequence 01101010 of a 10 Gbit s −1 DPSK signal at the input of a silicon CROW is shown by dashed curves, whereas the same sequence after wavelength conversion into the CROW over a wavelength range λ c − λ s of ( a ) 7 nm and ( b ) 49 nm is shown by the blue and red solid curves, respectively. The plots show the 10 Gbit s −1 intensity-modulated signal detected at the output of the Mach–Zehnder delay interferometer (see Methods ). The similarity between the input (signal) and output (converted) waveforms demonstrates that no significant phase information distortion occurs. Full size image Signal refurbishment The properties discussed above reveal that travelling-wave resonant FWM can be effectively exploited in all the applications where conventional FWM is employed, including, among others, the restoration of signal quality [36] . We exploited our silicon CROW to demonstrate signal retiming and reshaping in travelling-wave resonant regime. Time jitter and pulse broadening were induced on an intensity-modulated 10 Gbit s −1 non-return to zero (NRZ) data stream by propagation through 30 km of standard fibre. The propagation induces a root mean square (r.m.s.) 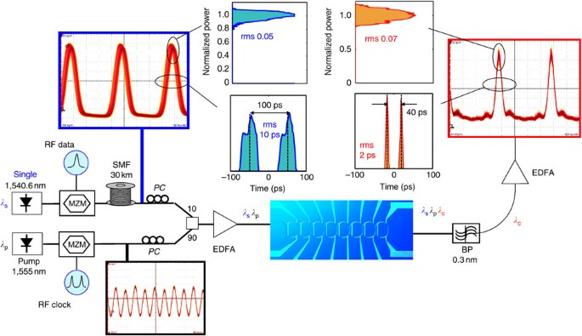Figure 7: Signal retiming via travelling-wave resonant FWM. The time jitter of an intensity-modulated 10 Gbit s−1NRZ data stream is reduced from 10 to 2 ps r.m.s. by exploiting wavelength conversion in a silicon CROW via FWM with a 10 GHz sinusoidal pump. Amplitude drift increases from 5% to only 7%. BP, bandpass filter; MZM, Mach–Zehnder modulator; PC, polarization controller; RF, radio frequency; SMF, standard single-mode fibre. fluctuation of the pulses time position of about 10 ps (corresponding to more than 40 ps peak-to-peak time drift) and an intensity jitter of the pulse peak of about 5% at the sampling instant, as shown in the histograms of Figure 7 . If a signal-synchronized pulsed pump wave is used in the FWM process, the jittered input signal undergoes a nonlinear 'sampling' effect that produces a retiming as well as a reshaping of the input pulse in the converted wave. Figure 7: Signal retiming via travelling-wave resonant FWM. The time jitter of an intensity-modulated 10 Gbit s −1 NRZ data stream is reduced from 10 to 2 ps r.m.s. by exploiting wavelength conversion in a silicon CROW via FWM with a 10 GHz sinusoidal pump. Amplitude drift increases from 5% to only 7%. BP, bandpass filter; MZM, Mach–Zehnder modulator; PC, polarization controller; RF, radio frequency; SMF, standard single-mode fibre. Full size image This retiming technique is transparent to both intensity- and phase-modulated RZ formats and operates a format conversion from NRZ into RZ signals. The converted signal has a residual r.m.s. time jitter of less than 2 ps. It is worth noting that the process is not just a gating mechanism and that the pulse shape is partially regenerated during the wavelength conversion. Using a sinusoidally modulated pump, the converted pulse shape is narrowed alongside the retiming effect, while the time jitter is partially converted into peak intensity fluctuations. This explains the slight increase (from 5 to 7%) observed in the intensity fluctuation of the converted signal; however, this effect is not related to the travelling-wave resonant FWM mechanism but is ascribed to the shape of the pump signal modulation that can be optimized to achieve the desired reshaping effect (time jitter suppression, format conversion, extinction ratio enhancement, etc.) [36] . Our results demonstrate that, besides conventional approaches based on the search for highly nonlinear materials [14] , [15] , [23] , [24] and on the design of optimally engineered waveguides [37] , [38] , there is a further level, namely the circuit level, that one can utilize to improve nonlinear interactions and that has been undervalued so far. Travelling-wave resonant propagation in CROWs is an effective way to fully exploit this option, leveraging performance improvement over non-resonant waveguides or lumped resonators. Besides enhancing the conversion efficiency, travelling-wave resonant propagation makes the FWM process particularly robust against the chromatic dispersion and the propagation loss of the waveguide, while entirely preserving the intrinsic transparency to modulation formats. Compatibility with a wide range of technological platforms enables the combination with alternative approaches based on optimized waveguide and material designs. The concept of travelling-wave resonant FWM can be extended to a much higher speed, as technologies providing up to 2 THz bandwidth resonators are already available [39] . This would enable exploitation of the full potential of all-optical processing and allow the manipulation of extremely broad bandwidth signals, well beyond the domain of electro-optics (>100 GHz). Device fabrication The CROWs were realized on a CMOS-compatible SOI wafer in the James Watt Nanofabrication Centre at the University of Glasgow by an optimized hydrogen silsesquioxane electron-beam-resist based fabrication process previously developed [40] . Light coupling was optimized through modal adapters realized by an inversely tapered section of the silicon wire, buried in an SU-8 polymer waveguide. The coupling coefficients of all the ring resonators are optimized by changing the gap distance between the rings in order to maximize transmission and reduce ripples within the CROW passbands [41] . Metallic NiCr/Au heaters, having a 900×50 nm 2 cross section and a total length of 54 μm, were deposited on the top of the waveguides and patterned by a lift-off technique for post-fabrication trimming of the device response. The heaters' geometry was designed not to overlap with the coupling regions between the ring resonators so as to minimize thermal crosstalk. Experimental setup for spectral characterization and device tuning The spectral characterization of the intensity response of silicon CROWs was obtained by an optical spectrum analyser (OSA) synchronized to a tunable laser source and controlled by a PC-based acquisition system. The polarization controller employed to calibrate the polarization state of input light guarantees an extinction ratio >35 dB between the launched TE and TM modes; spurious TM light coupled into the CROW is visible in the stop band of Figure 2b . Light coupling to and from the devices is achieved by microlensed tapered fibres (mode field diameter 1.7 μm) aligned to the SU-8 polymer modal adapters using nano-positioning stages with piezoelectric actuators and active feedback. Light coupling loss was estimated to be 5 dB per facet for TE polarization. Post-fabrication thermal tuning of the rings' resonance was realized by independently driving the metallic heaters deposited on the ring waveguides. A proprietary algorithm based on phase-sensitive low-coherence experimental characterization [42] of the devices was used to recover the optimal tuning parameters for each structure. Closed-loop Peltier thermocoolers were used for the temperature stabilization of the samples and thermal crosstalk between the ring resonators was observed to be negligible (about 1–2%) [25] . Experimental setup for FWM and time-domain measurements The pump signal used for the FWM experiments was amplified by an erbium-doped fibre amplifier (EDFA) with a maximum CW output power of 100 mW. The pump power coupled into the silicon waveguide was 12 dBm. The conversion efficiency of bare silicon waveguides was estimated by measuring several 5-mm ( P c / P s =−36 dB) and 10-mm-long ( P c / P s =−31 dB) waveguides fabricated on the same chip of the tested CROWs. The time traces shown in the time-domain measurements were acquired with a sampling oscilloscope (20 GHz electrical bandwidth) after the converted signal had been separated from the pump and the probe signals with a tunable optical filter (−3 dB bandwidth 0.3 nm) and then amplified using an EDFA with a low-noise figure. The 10 Gbit s −1 DPSK signal was generated by phase modulating a distributed feedback (DFB) laser through a commercially available lithium niobate modulator. After being wavelength converted by the CROW, the datastream was detected by an integrated Mach–Zehnder delay interferometer, unbalanced by 100 ps (1 symbol at 10 Gsym s −1 ) and realized in silicon oxynitride technology [43] . In the retiming/reshaping experiment, the launched power in the fibre was quite low, around 1 mW, to prevent any nonlinear effects. The time jitter occurs on a micro- and milli-second scale and it is induced by acoustic and thermal effect in the fibre spoil. After propagation, the incoming jittered signal is combined with a 10 GHz sinusoidally modulated pump wave and both are amplified as shown in Figure 7 . The modulated pump wave had a 3-dB modulation depth and a waveguide peak power of 40 mW (average power 30 mW). The two signals were time-synchronized by means of a glass tunable CROW delay line [26] to efficiently sample the jittered signal and obtain a reshaped replica at the converted wave. How to cite this article: Morichetti, F. et al . Travelling-wave resonant four-wave mixing breaks the limits of cavity-enhanced all-optical wavelength conversion. Nat. Commun. 2:296 doi: 10.1038/ncomms1294 (2011).